Microevolution ofNeisseria lactamicaduring nasopharyngeal colonisation induced by controlled human infection Neisseria lactamica is a harmless coloniser of the infant respiratory tract, and has a mutually-excluding relationship with the pathogen Neisseria meningitidis . Here we report controlled human infection with genomically-defined N. lactamica and subsequent bacterial microevolution during 26 weeks of colonisation. We find that most mutations that occur during nasopharyngeal carriage are transient indels within repetitive tracts of putative phase-variable loci associated with host-microbe interactions ( pgl and lgt ) and iron acquisition ( fetA promotor and hpuA ). Recurrent polymorphisms occurred in genes associated with energy metabolism ( nuoN , rssA ) and the CRISPR-associated cas1 . A gene encoding a large hypothetical protein was often mutated in 27% of the subjects. In volunteers who were naturally co-colonised with meningococci, recombination altered allelic identity in N. lactamica to resemble meningococcal alleles, including loci associated with metabolism, outer membrane proteins and immune response activators. Our results suggest that phase variable genes are often mutated during carriage-associated microevolution. Within-host selection of some bacterial species has been investigated in a variety of human niches during natural disease [1] . In the respiratory tract, startling levels of genomic change have been observed in pathogens during disease. Examples include diversifying hypermutation among Burkholderia dolosa populations [2] and convergent evolution in Pseudomonas aeruginosa sub-lineages, both among sufferers of cystic fibrosis [3] , [4] . At the gene-level, mutations within a small number of loci, mediating DNA mismatch repair systems, can lead to hypermutation among host-pathogen interaction genes [2] . Genetic diversity can also be caused by phase variation resulting from random slipped-strand mispairing in hypermutable, repetitive, polymeric sequences in ‘contingency loci’, such as the lipooligosaccharide biosynthetic genes [5] , [6] , [7] . These can drive host- or population-specific, selection bottlenecks [8] . The result of this is phenotypic and stochastic variation in both colonisation and disease outcomes, which is enhanced by the acquisition of beneficial genetic material from unrelated organisms through the various mechanisms of horizontal gene transfer [9] . Colonisation is an important prerequisite for disease [6] , but beyond species-species interactions and clearance, very little is known about how colonising species are impacted by the cumulative challenges experienced when occupying a new niche. Asymptomatic carriage of Staphylococcus aureus in the anterior nares is associated with rare adaptive change, but invasive isolates exhibit very little genomic variation compared to carriage isolates [10] , [11] . Regarding the nasopharyngeal pathogen Neisseria meningitidis , a study contrasting bloodstream and nasal isolates from four individuals found no evidence of gene-specific convergent evolution but detected phase variation in type IV pilus biogenesis loci [12] . Neisseria lactamica is an exclusively human nasopharyngeal commensal with highest prevalence of carriage in infancy. Carriage of N. lactamica has an inverse epidemiological relationship with infections caused by N. meningitidis [13] . Here, we used two controlled human infection studies to examine the microevolution of N. lactamica , a harmless commensal, genetically and phenotypically similar to N. meningitidis and Neisseria gonnorhoeae [14] . Initially, a short-term colonisation study was used to contrast N. lactamica collected from in vivo and in vitro passage over a period of 1 month. A second study, the purpose of which was to explore the potential, protective effect of N. lactamica colonisation in young adults, a demographic at risk of Neisseria infection [15] , examined inoculated N. lactamica , other wild-type N. lactamica and wild-type N. meningitidis collected [16] , over 6 months of carriage. In this work, we determine the intra-host genomic diversification of N. lactamica over time, comparing this with in vitro dynamics. We contrast the contribution of non-synonymous polymorphisms to that of mutations in contingency loci that drive phase variation. In addition, we examine the frequency of recombination, inferring horizontal gene transfer (HGT) events between both inoculated and wild-type N. lactamica with N. meningitidis . Using estimates of diversity, we determine the effective population size in colonised individuals. These results offer insights into the impacts on genomic structure and micro-evolutionary processes in a bacterial coloniser of the human respiratory tract. 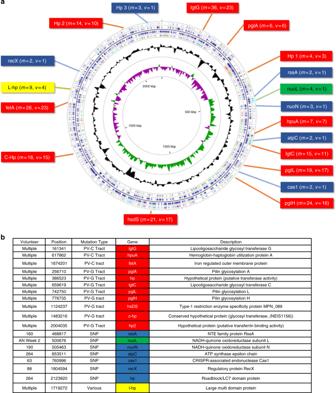Fig. 1 a,bMutations that occurred in isolates recovered over 6 months of nasopharyngeal carriage are outlined as follows: changes to repetitive tracts of phase-variable, contingency loci (Red), genes in which SNPs were persistently detected across multiple volunteers (Blue), including an example from the short-term, in vitro VS in vivo study (Green) and the sole gene in which various mutations discovered across multiple timepoints and volunteers (Yellow).mrefers to the number of mutations detected in a given gene acrossvvolunteers. The genes are placed in positions relative to their approximate location in theN. lactamicaY92-1009 genome.bVolunteers in which Single-Nucleotide Polymorphisms (SNPs) were seen are specified in the Volunteer column. Mutations which affected multiple volunteers are quantified in the accompanying figure above. Mutation locations are indicated in the Position column. The type of mutation is given in the mutation column where C tract/G tract refers to a homopolymeric region of cytosine/ guanine repeats where insertions and deletions occurred. PV denotes phase-variable Mutations and effective population size We recovered isolates from throat swabs taken from volunteers who had been inoculated with 10 4 CFU ml −1 of N. lactamica Y92–1009 cell bank stock [17] for a short period (1 month) of carriage and compared them with isolates that underwent in vitro passage for the same period of time (Supplementary Figure 1 ; additional data in Supplementary Data 1 ). Isolates that had undergone passage in vitro exhibited a greater number of non-synonymous and stop codon single nucleotide polymorphisms (SNPs). There were also more insertions ( n = 6 base insertion events) observed during in vitro passage. Isolates from colonised participants had marginally more synonymous SNPs but no insertions, only one deletion and no SNPs introducing premature stop codons. Deleterious mutations observed in the in vitro isolates involved citrate synthase ( gltA) and pilin subunit ( pilP ) genes and, once fixed in the population, were seen to recur in all subsequent isolates. This contrasts with isolates recovered from volunteers who had undergone controlled infection (ie in vivo), in which almost all SNPs occurred only once per sampling point despite multiple colony sampling. Mutations in mqo (Malate:quinone oxidoreductase) and phrB which confers resistance to nalidixin and rifampicin in N. gonorrhoeae [18] , were seen to occur in both datasets; however, the position of mqo mutations differed while the synonymous phrA mutation occurred in the same position in both the in vitro controls as well 2/5 colonised volunteers (Supplementary Data 1 ) A greater number of mutations in genes containing hypermutable, polymeric tracts, i.e. phase variable genes, were observed in vivo. These were compared to those identified in vitro over a month. No unique in vitro mutations were identified (i.e. these were also seen in vivo); conversely, novel in vivo changes in repetitive sequences were observed. Two of these genes were primarily associated with the modification of lipooligosaccharide(LOS), known to mediate host-pathogen response (glycosyltrasnferases; lgtG gene). There was also phase variation detected in the specificity subunit ( hsdS ) of the type 1, dual gene, NgoAV restriction modification system and genes implicated in iron acquisition among Neisseria spp. ( hpuA and rubredoxin). Phase variation was also observed in a conserved hypothetical protein with putative glycosyl transferase activity (Table 1 ). No consistent pattern of phase switching ON vs phase switching OFF was observed among the isolates tested (Supplementary Data 2 ), however, two genes, the haemoglobin receptor hpuA and glycosy ltransferase lgtG exhibited a significant shift from PHASE ON - > OFF in weeks 8 and 4 respectively (< p = 0.05 Fisher’s exact test). Table 1 Phase-variable locus mutations observed in comparison of in vitro passage and in vivo colonization during short-term carriage (1 month) Full size table Substitution rate estimates were five times greater in the in vitro isolates (7.55 × 10 −5 substitutions per site per year) compared to the in vivo isolates (1.45 × 10 −5 substitutions per site per year, extrapolated from 1 month of carriage). Tajima’s D, a comparison of pairwise differences and segregating sites in a given population of alleles, was used to indicate whether the population was undergoing positive (selective sweeps) or negative selection. 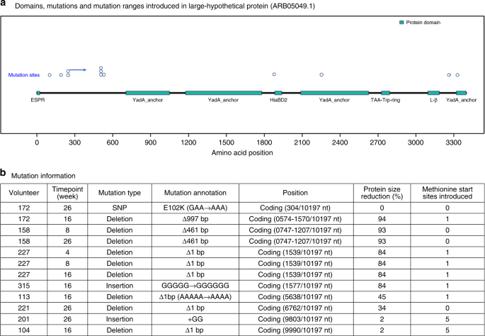Fig. 2 Domains, mutations and mutation areas of effect introduced in Large-Hypothetical Protein (ARB05049.1) (a) with the distribution found between volunteers (b). Mutations are coloured blue and white and are listed inbin the order they occur along the protein depicted ina Here the statistic was negative (approximately −1) for both in vivo and in vitro (Table 2 ), an indication of selective sweeps and a function of rare mutations in the population. Additionally, the estimates of effective population size ( N e ) were low (~18) and approximately the same for both sample sets. Whilst differences appeared in both the rate and type of mutation that occurred during in vivo colonisation, as compared to in vitro passage, the overall impact on population genomic diversity was similar. Table 2 Effective population size and Tajima’s D calculated for N. lactamica Y92–1009 sample sets Full size table Microevolution during long-term N. lactamica carriage in humans In a controlled human infection model, in which 149 volunteers were inoculated with N. lactamica intranasally, a total of 95 isolates of N. lactamica Y92–1009 and 14 isolates of N. meningitidis from 37 participants recovered over 6 months [16] were sequenced. An additional two individuals carried wild-type N. lactamica belonging to sequence types other than the inoculum strain (ST-4192 and ST-11524, n = 9 isolates) and are discussed later. In 91% ( n = 32) of participants, N. lactamica was isolated from more than one sampling point over the course of 6 months. In 8 individuals both N. lactamica and N. meningitidis were isolated, with 4 individuals having simultaneous carriage of both species. A total of 268 mutations were identified in N. lactamica following isolation. The most prevalent (71.6%, n = 192), were modifications to repetitive tracts in putatively phase variable loci. A list of genes containing 6–14 nucleotide homopolymeric tracts in the N. lactamica Y92-1009 are detailed in Supplementary Data 3 . From this list of 98 genes, 11 contingency loci were found in which phase variation recurred longitudinally, within and between volunteers (Fig. 1a, b ). All contingency loci were found to contain homopolymeric G/C tracts, despite evidence of A/T tracts among the 98 candidate loci. Genes affected by these mutations were involved in LOS and pilin subunit modification ( lgt and pgl loci), iron acquisition ( hpuA ) and type I restriction-modification ( hsdS ). The hypothetical proteins were assigned putative function as glycosyl transferases (hp and c-hp), and transferrin binding activity (hp2). While most of these mutations occurred in polymeric tracts located within coding sequence, 28/192 were detected in an intergenic promotor region bordering the fetA gene, potentially modulating transcriptional efficiency. All isolates contained changes in the repeat tracts of at least two of these contingency loci. Fig. 1 a , b Mutations that occurred in isolates recovered over 6 months of nasopharyngeal carriage are outlined as follows: changes to repetitive tracts of phase-variable, contingency loci (Red), genes in which SNPs were persistently detected across multiple volunteers (Blue), including an example from the short-term, in vitro VS in vivo study (Green) and the sole gene in which various mutations discovered across multiple timepoints and volunteers (Yellow). m refers to the number of mutations detected in a given gene across v volunteers. The genes are placed in positions relative to their approximate location in the N. lactamica Y92-1009 genome. b Volunteers in which Single-Nucleotide Polymorphisms (SNPs) were seen are specified in the Volunteer column. Mutations which affected multiple volunteers are quantified in the accompanying figure above. Mutation locations are indicated in the Position column. The type of mutation is given in the mutation column where C tract/G tract refers to a homopolymeric region of cytosine/ guanine repeats where insertions and deletions occurred. PV denotes phase-variable Full size image Transient SNPs in non-phase varying genes were the second most abundant mutations (46/268, 17%). These occurred after various intervals within different volunteers and were detected once. A total of 29 non-synonymous SNPs, 15 synonymous SNPs, 3 insertions, 2 multiple base substitutions and 3 deletion events were observed (Supplementary Data 4 ). We defined a persistent mutation as one which was identified in consecutive isolates. A total of 15 SNPs, disseminated among five of the volunteers, were found to persist longitudinally. These were found in lipid-hydrolase protein rssA , oxidoreductase nuoN , energy synthase atpC and CRISPR-associated endonuclease cas1 and two hypothetical proteins. In addition to this, seven deletion events appeared fixed in three volunteers, these affected a large hypothetical protein and are discussed later in this section. The non-synonymous mutation found in rssA has been seen in another N. lactamica isolate found via BLASTp against the nr database. The location and nature of the remaining mutations were not identified in either sequence database blast of the entire catalogue of pubMLST Neisseria or via non-specific BLASTp against the nr database. Therefore, these are most likely novel polymorphisms found during the course of this study. These persistent mutations were shown alongside the phase variations in Fig. 1a, b and tabulated in Supplementary Data 5 . Convergent mutation was rare in this dataset; however, twelve mutations were found in eight (27%) of the volunteers that localized to a single, large (~10 kb) hypothetical protein (herein referred to as L-hp, accession: ARB05049.1) (Fig. 2 ). The sequence of this gene is specific to this strain and not detected outside of N. lactamica Y92-1009 in a sequence search among all Neisseria isolates in the pubMLST.org/neisseria database or non-specific BLASTp against the nr database. The locus is located at position 1,719,272 in the N. lactamica Y92-1009 genome, with a GC content (31.3%) that was skewed negatively, compared to the overall GC content of the genome (52.2%) closer towards the mean GC content for Haemophilus influenzae (~G + C: 38%). This was the only coding sequence devoid of phase variable tracts found to be targeted by mutation across multiple volunteers. L-hp contained 8 conserved protein domains which included an extended signal peptide of the type V secretion system (pfam13018), A tryptophan-ring motif (pfam15401), supporting a HiaBD2 trimeric autotransporter adhesin (pfam15403), Yad-A like, left-handed beta roll (cl17507) and four YadA-like C terminal regions (3 copies of cl27224 and pfam03895). Five of the twelve mutations persisted in volunteers 158 and 227, reducing the predicted protein size by 84–93%. Only two of the twelve mutations identified were seen to occur within the domains and both targeted YadA-like C terminal regions. CDART analysis, which contrasts the positions and functions of protein domain architecture but not necessarily sequence similarity, revealed significant homology with other N. lactamica strains (score = 5/5, three sequences) and H. influenzae (Mean GC content: ~38, score 4/5, thirteen sequences) and Neisseria cinerea ATCC 14685 hep/hag repeat protein (score = 4/5, two sequences) but only marginal or non-existent matches to other members of the Neisseriaceae . This indicates that three other N. lactamica strains possess this exact protein architecture (with regards to domain dissemination and function throughout the protein) with all five domains present, but that fifteen sequences from both H. influenzae and N. cinerea genomes possess proteins with very similar domain architecture. Protein BLAST analysis identified significant matches (>95% identity) only among other N. lactamica Y92-1009 genomes. Fig. 2 Domains, mutations and mutation areas of effect introduced in Large-Hypothetical Protein (ARB05049.1) ( a ) with the distribution found between volunteers ( b ). Mutations are coloured blue and white and are listed in b in the order they occur along the protein depicted in a Full size image Effect of recombination ClonalframeML was used to detect loci in N. lactamica affected by recombination in the core genome ( n = 1595 core loci) and to quantify the total effect of recombination compared to mutation (r/m) (Table 3 ). A total of 18 loci were detected as recombinant over the course of this analysis (Table 4 ). Three of these loci affected by recombination were identified in volunteers ( n = 27 volunteers) carrying only N. lactamica Y92-1009. These included a hypothetical protein (NEIS1708, NMB0444), a putative mafs3 cassette (NEIS1794) and an intracellular septation protein (NEIS1828, NMB0342). The effect of recombination (r/m) was 3.62, based on all volunteer isolates experimentally challenged with N. lactamica Y92-1009. Eight volunteers co-carried the experimentally inoculated N . lactamica Y92-1009 strain, however isolates from one volunteer were excluded from recombination analysis as only one isolate from N. meningitidis and N. lactamica was recovered leaving seven volunteers ( n = 19 isolates) with wild-type N. meningitidis (Table 3 ). Here the average r/m value was 3.84, which was similar to that seen when the bacterium was not co-colonised with N. meningitidis . Only small (<20 bp) importations were detected in volunteers co-carrying experimentally inoculated N. lactamica Y92–1009 and N. meningitidis . As a result, there were no recombinant loci identified in co-colonised individuals who were experimentally inoculated with N. lactamica . Table 3 Relative recombination effect (r/m) of isolates in colonised volunteers and the parameters used to infer them Full size table Table 4 Genes undergoing recombination Full size table Mutation rates and effective population size Given the above mutation parameters we estimated the effective population size for the N. lactamica inoculum. We inferred a mutation rate in terms of SNPs per site per year. Sixty-four SNPs were detected among twenty-seven volunteers carrying only N. lactamica Y92–1009. This yielded a mutation rate of 2.21 × 10 −6 substitutions per site per year. Seven SNPs were detected among seven volunteers co-colonised with N. meningitidis and were used to infer a mutation rate of 9.32 × 10 −7 substitutions per site per year. Therefore, no evidence of an enhanced mutation rate was observed in volunteers co-carrying the inoculated N. lactamica and strains of N. meningitidis . Tajima’s D was found to be negative (approximately −1) for N. lactamica isolates examined with or without meningococcal co-colonisation (Table 2 ). The estimations of effective population size ( N e ) were found to be consistently low in all four sets (Table 2 ). Recombination between co-colonising N. lactamica and N. meningitidis Two volunteers (36 and 291) were found to co-carry naturally acquired N. lactamica (ST-4192 and 11524, n = 9 isolates) in addition to commensal N. meningitidis (ST-41 and ST-10457, n = 6 isolates) (Supplementary Table 1 ). Together, these volunteers accounted for the majority of recombinant loci detected ( n = 15/18 loci, Table 4 ). Volunteer 255 was the only individual who was observed to carry more than one N. meningitis ST during this period: a-ST-10478 meningococcus at the first sampling point, followed by a ST-213 N. meningitidis . In contrast to the N. lactamica Y92-1009 challenge strain, the r/m values were between 3–5 times higher for wild-type N. lactamica and N. meningitidis (Table 3 ). The largest r/m (overall effect of recombination calculated as described in Table 3 legend.) detected was 18.06 and was calculated for volunteer 291 wild-type N. lactamica and may imply the organism was subject to a recent, interspecific recombination event although it is impossible to verify whether the event occurred before or during the course of the study. Six recombinant alleles were identified in the N. lactamica isolated from volunteer 291 that were also found in the co-carried N. meningitidis (Supplementary Figure 2 ). Of these six alleles, four (NEIS0071, a putative lipoprotein; NEIS0072 & NEIS2514, hypothetical proteins; and NEIS0899, lst , a LOS subunit sialyltransferase) were shared by N. lactamica and co-colonising N. meningitidis recovered from the second and third sampling points. By week 16 however a different allele for these loci was identified in the recovered N . lactamica . In contrast, for two loci (NEIS1834, an acyl carrier protein and NEIS1835, a succinyltransferase) it was the week 16 isolates that were found to share the same allele as the meningococci. This might suggest that these recombination events reflect independent exchanges, however this is not possible to determine from this data alone. As anticipated from previous in vitro studies of the meningococcus [19] , phase variation was the principle mechanism by which microbial diversity arose in the commensal carried by individuals over 6 months. With the assumption that the mutation rate estimate acquired from the largest number of volunteers (n = 97) over the longest period (26 weeks) is the most accurate, the value of 2.21 × 10 −06 substitutions per site, per year is in agreement with estimates detected in N. gonorrhoeae [20] , [21] , [22] and N. meningitidis [23] . Our values for effective population size in the four sample sets (long-term carriage of N. lactamica with and without co-carriage of N. meningitidis ; short-term carriage in vivo; in vitro passage) were much lower ( N e = 1–25) than those recently described among Escherichia coli examined over a year [24] , but comparable to those observed in Vibrio cholerae [25] . These latter two studies, however, examined different organisms in different niches, with the Vibrio observations collected during acute infection. A low effective population size may indicate the presence of severe bottlenecks or growth limitation, and our observations may be an outcome of the dynamic antagonistic and commensal processes that occur among members of the microbiota of the upper respiratory tract [26] . It is worth noting, too, that, at least in murine models of pneumococcal colonisation, N e was also found to be low, between 11 and 203, and thus comparable to our findings [27] , [28] . Although these numbers are derived from single colony isolates, and thus may not reflect the true genomic heterogeneity of the population [29] the low number of mutations observed longitudinally within individuals suggests the estimation of both mutation rate and Ne are accurate. Moreover, a similar substitution rate of 1.45 × 10 −5 SNPs per site per year was observed when multiple colonies were sampled among six volunteers in the short-term study (1 month), this is in contrast to the finding of a substitution rate of 2.21 × 10 −6 SNPs per site per year in the long-term study (6 months) across many more volunteers, albeit over a much shorter period of colonisation. Additionally, the bulk (70%) of the mutations observed in the short term in vivo (Supplementary Data 1 ) cohort occurred once per colony sampled. Mutation prevalence over all colonies at a given time point and mutation recurrence across time points were observed to be rare events. Purifying selection acts to remove non-beneficial mutations, and our observation that most SNPs were transient, non-recurrent events, combined with a negative Tajima’s D value, suggest that diversity was lower than expected, consistent with the population being subject to bottleneck events. Despite this, some non-synonymous SNPs persisted longitudinally in some volunteers, becoming fixed in the sample and staying for at least one further time point. These included non-novel mutations in rssA and novel mutations in the nuoN , rssA , 2 hypothetical proteins and cas1 loci. The nuo operon, which encodes subunits for NADH dehydrogenase complex I, is among those genes upregulated in iron replete conditions in N. gonnorhoeae [29] and N. meningitidis incubated in human blood [30] . Cas1 acts as a dsDNA endonuclease in a minimal, self-promoted, CRISPR-Cas type II-C system in N. lactamica , that has been postulated to provide adaptive protection to its host from unbeneficial, exogenous, horizontal gene transfer [31] . The persistent mutations in phospholipase RssA represent the first evidence of this gene adapting to the oropharyngeal environment. Most of the insertion and deletion events not present in contingency loci affected one gene: a large, (~10,000 bp) multi domain hypothetical protein (L-hp). An in-silico simulation of how these mutations might affect protein coding revealed frame-shifted introductions of interproteomic methionine residues and overall reductions in predicted protein size. The L-hp locus was the only region in which mutations were seen to persist in some volunteers. The low GC content of this locus relative to N. lactamica Y92-1009 suggests that it may have been horizontally acquired by N . lactamica from another nasopharyngeal coloniser, perhaps H . influenzae , based on the results from CDART and the possession of a H . influenzae autotransporter domain. This is not uncommon and there are other examples of genes postulated to have been acquired by N. lactamica 020-06 from H. influenzae , including phosphroylcholine biogenesis genes licABCD , ATPase gene slpA , protease gene slpB and putative surface fibril protein NLA12600 [32] . The presence of trimeric autoadhesins such as the YadA -like and Hia conserved domains, suggest this protein may have a role in initial attachment of the bacterium to a human host [33] . Post-colonisation, it may be that the deletion of these proteins is beneficial, perhaps metabolically or as it is a site for host-recognition. In conclusion, N. lactamica Y92–1009 possesses a stable genome that undergoes stochastic mutation, at a low mutation rate with minimal evidence of recombination or interspecific interaction with co-colonising meningococci, as was demonstrated by wild-type N. lactamica . However, the observed genetic changes indicate an important role of phase variation among genes associated with host-commensal interaction and iron acquisition in sustained colonisation of human hosts. A lack of microevolutionary evidence in N. lactamica isolates co-colonised with N. meningitidis suggests that the meningococcal carriage suppression induced by N. lactamica may be due to outcompeting the pathobiont for essential resources in the nutrient-limited, nasopharyngeal niche. Controlled human infection with N. lactamica N. lactamica Y92–1009 was originally isolated during a 1992 carriage study of school pupils in Londonderry, Northern Ireland. Its use in an experimental human challenge model (Clinical Trial Registration: NCT02249598) has been reported previously [16]. The study was approved by the National Health Service Research Ethics Committee (11/YH/0224), was overseen by an independent safety committee, and was conducted in accordance with the Declaration of Helsinki. Written informed consent was gained from participants prior to inclusion in the study. Briefly, 149 participants received nasal challenge with 10 4 CFU of N. lactamica . In this group, natural N. meningitidis carriage at baseline was 36/149 (24.2% [95% CI, 17.5%–31.8%]). Natural carriage of N. lactamica prior to inoculation was observed in 3/149 individuals (1.9% [95% CI, .4%–3.5%]). Following challenge, oropharyngeal swabs were taken at 2, 4, 8, 16, and 26 weeks and were plated directly onto gonococcus (GC)-selective media (E&O Laboratories, Scotland) and incubated at 37 °C in 5% CO 2 . After 48 hours, possible Neisseria spp. colonies were subjected to API-NH strip testing (bioMérieux, France) and PCR [16] . The isolates were not extensively passaged. Growth was limited to two passages (one for isolation from the host and one for preparation of sequencing). Two weeks after inoculation, oropharyngeal swabs from 48 individuals challenged with N. lactamica yielded cultivable N. lactamica (33.6% [95% CI, 25.9%–41.9%]), but colonization with N. lactamica was detected as late as week 26, by which time colonisation with N. lactamica at some point in the study had been confirmed in 61 of 149 (41.0% [95% CI, 33.0%–49.3%]) of the challenge group. All isolates of N. lactamica and N. meningitidis were cryostored. The study flow is summarised in Supplementary Figure 3 . Choice of Neisseria isolates for genomic analysis The inclusion strategy prioritised the following: (a) isolates from individual volunteers that were recovered from multiple sampling points; (b) isolates from volunteers co-colonised with N. meningitidis ; and, (c) isolates recovered either early (week 2) in the study or later (week 26), with the rationale that the isolates from earlier time points had undergone adaptation and selection more recently and the isolates at the late time point would have a greater chance of demonstrating signs of convergent evolution, having colonised their respective hosts for the longest period of time. In total 97 N. lactamica Y92–1009, 14 N. meningitidis and 9 non-Y92–1009 N. lactamica isolates were chosen for sequencing and analysis. These isolates are summarised in Supplementary Data 6 Comparison of in vitro passage vs. in vivo colonisation To compare stochastic mutation during in vitro passage with variation observed intra-host, 10 additional volunteers were intra-nasally inoculated with 10 4 CFU ml −1 N. lactamica Y92–1009 stock. Oropharyngeal swabs were used to take samples at days 1, 2, 3, 14 and 28. Colonisation was established in five of the ten volunteers. In vitro serial passages were done in duplicate and in parallel with the in vivo colonisation study. Isolates, consisting of 1–5 colonies, were subcultured on Columbia blood agar every weekday for 28 days. A maximum of five colonies of N. lactamica from each sampling point were selected and sequenced. Culture Bacterial samples were recovered from cryostorage (−80 °C) and streaked onto Columbia + horse blood plates and cultured overnight at 37 °C. N. lactamica colonies were confirmed using X-gal (Sigma Aldrich, USA) in PBS. Two blue colonies were then subcultured into bijoux tubes, each containing 2 ml Tryptic Soy broth with 0.2% yeast extract (Sigma Aldrich, USA). The cultures were grown overnight with agitation at 37 °C. Genomic DNA extraction Genomic DNA was extracted using the Wizard Genomic Purification Kit (Promega, USA). Sample purity and concentration (OD 260/280) were assessed using a Nanodrop 1000 spectrophotometer (ThermoFisher, UK) and Qubit 2.0 fluorometer with the BR dsDNA kit (Invitrogen, UK). For long read sequencing of the reference genome, a sample of cell bank purified stock was cultured and extracted using the Gentra Puregene yeast/bacteria kit according to manufacturer’s instructions (Qiagen, Germany) to produce 30 µg of high molecular weight (>40 kDA) DNA. Sequencing All isolates of N. lactamica were sequenced using an Illumina HiSeq 2000 instrument as described previously [34] to generate 2 × 151 bp PE libraries. For the reference genome, high molecular weight DNA was pooled and sequenced using the Pacific Biosciences RSII instrument as outlined in [17] (Earlham institute, Norwich). Data for the reference strain is available on NCBI with accession CP019894. Genome assembly, correction and annotation Reads were assembled using velvet optimiser and added to the PubMLST Neisseria database [35] [ https://pubmlst.org/neisseria/ ]. The resultant contigs were annotated using automated processes to identify specific loci using the PubMLST.org/neisseria ‘NEIS loci’ catalogue [36] The reference genome was assembled at the Earlham institute (as described in [17] ). Error correction of the reference was done with Illumina reads using Pilon v1.17 [37] . Annotation was done using Prokka v1.11 [38] aided by a curated protein list from N. lactamica 020-06 (accession: FN995097). Mutational and recombination analyses Mutational analysis was performed by mapping reads against the reference genome assembly using the breseq v0.23b pipeline [39] . In addition, in order to determine the novelty of persistent, volunteer-specific, and in one case, non-specific non synonymous mutations identified in this study, the specific location and amino acid changes relative to that position of mutants were searched via sequence database BLAST of the entire Neisseria loci catalogue hosted on pubMLST Neisseria database and via non-specific BLASTp against the nr database. Recombination analysis was done using ClonalFrameML v1.25 (CFML) [40] using core XMFA alignments and a core genome, maximum-likelihood (ML) tree as input. The genome comparator tool [ https://pubmlst.org/neisseria/ ]was used to determine core NEIS loci. Before generating an alignment, the NEIS loci were exported in FASTA format and screened for paralogues using CD-HIT v4.6.6 [41] which were excluded from the pool of core NEIS loci. The genome comparator tool was then used to output core XMFA and FASTA alignments, the former to be used as input to CFML, the latter to be used to construct a ML tree. The ML tree was created by converting the FASTA alignment to PHYLIP format using EMBOSS seqret v6.6 [42] and running PHYML v20131022 [43] on the PHYLIP alignment using the HKY85 model. This process also outputted a transition/transversion ratio to be used as the -kappa input parameter in CFML. ML trees were converted to binary format using the R package ape v3.0 [44] . The use of XMFA files with CFML introduced 1000 bp spacer segments between each gene in the alignment. The subsequent data on the location of recombinant alleles was adjusted to correctly confirm their identity. Any recombinant alleles were examined manually using mView [45] to confirm significant divergence suggesting recombination instead of false positives due to interspersed, minor mutation events. Phase variation ON VS OFF statistics Six genes, lgtG , lgtC , pglA , pglH , hsdS and hpuA were tested for significant differences in phase ON vs phase OFF status in weeks 2, 4, 8, 16 and 26. These six were tested as we limited the analysis to those that underwent at least one phase variation and where putative ON/OFF expression status data was available in the literature from other Neisseria spp. [46] , [47] . In addition, fetA was excluded as this is not an ON/OFF phase variable event but a promotor-dependent modulator for transcriptional efficacy, the role of which is unconfirmed in this Neisseria spp. Fishers exact tests using 2 × 2 contingency tables were tested in GraphPad Prism contingency table calculator [48] . The input into the table was the number of isolates for an early time point which had putative phase ON copy numbers vs putative phase OFF copy numbers. The second row of the contingency table contains the isolates with ON/OFF copy number for the later time point to be tested. When testing isolates in week 2, null values were used in place of week zero samples in the contingency table. Protein sequence analysis Where applicable, hypothetical proteins were investigated using the conserved domain architecture tool [49] , which was used to meta-analyze the predicted protein domains. These domains, alongside any mutations that were seen to occur during longitudinal carriage, were used as input for plot protein [50] to generate a protein diagram. In silico translations to determine effects of mutation on protein size were examined using ExPASy translate [51] . Effective population size, selection and mutation rate calculations Core loci alignments, generated as described above, were used as input for the R package PopGenome [52] to test for selection using Tajima’s D [53] and to calculate diversity via Tajima’s theta ( θ ). The mean values for Tajima’s D and θ were taken and the standard deviation of the population was calculated. Mutation rate ( m ) was calculated as the number of SNPs per site per year. Effective population size ( N e ) was estimated by rearranging the formula θ = 2 gN e mL to N e = θ / (2 mgL ) [54] , where θ is the mean genetic diversity using Tajima’s theta, m is the mutation rate per site per year, g is the generation rate (estimated to be roughly one cell division per day: 1/365) and L is the genome length (2,146,723 bp).